Evidence of indirect gap in monolayer WSe2 Monolayer transition metal dichalcogenides, such as MoS 2 and WSe 2 , have been known as direct gap semiconductors and emerged as new optically active materials for novel device applications. Here we reexamine their direct gap properties by investigating the strain effects on the photoluminescence of monolayer MoS 2 and WSe 2 . Instead of applying stress, we investigate the strain effects by imaging the direct exciton populations in monolayer WSe 2 –MoS 2 and MoSe 2 –WSe 2 lateral heterojunctions with inherent strain inhomogeneity. We find that unstrained monolayer WSe 2 is actually an indirect gap material, as manifested in the observed photoluminescence intensity–energy correlation, from which the difference between the direct and indirect optical gaps can be extracted by analyzing the exciton thermal populations. Our findings combined with the estimated exciton binding energy further indicate that monolayer WSe 2 exhibits an indirect quasiparticle gap, which has to be reconsidered in further studies for its fundamental properties and device applications. Two-dimensional (2D) transition metal dichalcogenides (TMDs) in the family of MX 2 (M:Mo, W; X:S, Se) have been discovered as a new class of semiconductors for atomically thin electronics and optoelectronics [1] , [2] , [3] , [4] , [5] , [6] . Of particular interest are monolayer MX 2 , which have been identified as direct gap semiconductors and emerged as new optically active materials for developing novel 2D light emitters and absorbers [5] , [6] . Experimental evidence of direct gap in monolayer MX 2 was obtained from the observation of strongly enhanced photoluminescence (PL) caused by the indirect to direct gap transition when MX 2 were thinned to one monolayer [7] , [8] . Although most theoretical calculations have also shown a direct gap at K-valley in all monolayer MX 2 [9] , [10] , [11] , [12] , subtle differences have been found in some calculations for monolayer WSe 2 [13] , where the conduction band (CB) minimum lies at Q-valley (about midway between K and Γ). Indeed, recent scanning tunneling spectroscopy (STS) suggested that the Q-valley is about 80 meV below the K-valley in the CB of monolayer WSe 2 [14] , indicative of an indirect quasiparticle gap. However, due to the unusually strong Coulomb interactions and the lack of knowledge on the binding energy of indirect excitons, it remains unclear whether the optical gap (i.e., quasiparticle gap minus exciton binding energy) is also indirect. While efficient PL is invariably observed in monolayer WSe 2 , the indirect quasiparticle gap observed by STS suggested that the direct/indirect nature of optical gap in monolayer WSe 2 has not been settled thus far. Strain is an effective perturbation that can modulate not only the direct gap of MX 2 , but also the indirect gap with a different trend [11] , [15] , [16] , [17] , [18] . As the indirect gap energy is pushed away from or brought closer to the direct gap by strain, the exciton population participating in the direct-gap recombination will be affected by the presence of nearly degenerated indirect gap, leading to a modulation in the energy and intensity of direct exciton PL. In this work, instead of applying external stress, we investigate the spatially resolved PL from monolayer WSe 2 –MoS 2 and MoSe 2 –WSe 2 lateral heterojunctions (HJs) with inherent nonuniform strain distribution [19] . The built-in local strain inhomogeneity exhibited in lateral HJs provides a unique platform to study the strain effects on MX 2 without the need of applying strain. Here we first demonstrate PL from strained MoS 2 in WSe 2 –MoS 2 lateral HJs as a model system to extract the energy difference between the direct and indirect gaps in monolayer MoS 2 . Then we demonstrate the study of MoSe 2 –WSe 2 lateral HJs and show that unstrained monolayer WSe 2 is actually an indirect gap material. 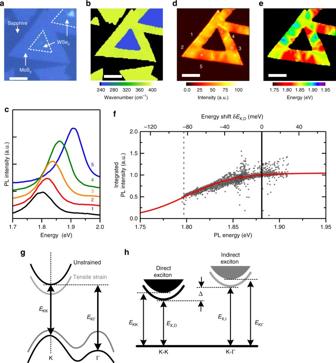Fig. 1 PL inhomogeneity in strained WSe2–MoS2lateral HJs.a,bOptical image (a) and the corresponding contour color map of the E2gRaman peak position (b) of a monolayer WSe2–MoS2lateral HJ flake.cFive selected PL spectra from different positions in the MoS2region.d,eContour color maps of the PL intensity (d) and peak energy (e) of the MoS2region.fIntegrated PL intensity as a function of peak energy obtained from all PL spectra (black dots). Solid line is the model fitting curve. The top axis is the PL peak energy shift with respect to the unstrained MoS2(vertical line).gSchematics for the band structures of monolayer MoS2without (black) and with (gray) tensile strain.hSchematics for the direct (K-K) and indirect (K-Γ) excitonic states with energies ofEX,DandEX,I, respectively PL inhomogeneity in strained WSe 2 –MoS 2 lateral HJs Figure 1a shows the optical image of a typical WSe 2 –MoS 2 lateral HJs. Raman analysis (Fig. 1b ) reveals that the inner and outer regions are monolayer WSe 2 and MoS 2 , respectively. The typical size of the HJ flakes is ~ 15–25 μm. According to ref. [19] , the outer MoS 2 exhibits nonuniform strain distribution due to the lattice mismatch between two materials, leading to considerable spatial variations in local PL spectra in the outer MoS 2 . Figure 1c shows five selected PL spectra, of which the PL energy variation is ~ 100 meV, corresponding to a strain variation up to ~ 2% in the monolayer MoS 2 (based on the reported linear PL energy shift rate of ~ 45 meV/% strain) [16] . As shown in Fig. 1d and e , the spatial distributions of PL intensity and energy in outer MoS 2 show a “positive” correlation, i.e., the site with a higher PL energy always exhibited a higher intensity. The PL intensity–energy correlation can be seen clearly in Fig. 1f , where the integrated intensities and peak energies collected from all local PL spectra of the outer MoS 2 are plotted together. Fig. 1 PL inhomogeneity in strained WSe 2 –MoS 2 lateral HJs. a , b Optical image ( a ) and the corresponding contour color map of the E 2g Raman peak position ( b ) of a monolayer WSe 2 –MoS 2 lateral HJ flake. c Five selected PL spectra from different positions in the MoS 2 region. d , e Contour color maps of the PL intensity ( d ) and peak energy ( e ) of the MoS 2 region. f Integrated PL intensity as a function of peak energy obtained from all PL spectra (black dots). Solid line is the model fitting curve. The top axis is the PL peak energy shift with respect to the unstrained MoS 2 (vertical line). g Schematics for the band structures of monolayer MoS 2 without (black) and with (gray) tensile strain. h Schematics for the direct (K-K) and indirect (K-Γ) excitonic states with energies of E X,D and E X,I , respectively Full size image The PL intensity–energy correlation arises from the variation of direct exciton populations caused by the strain-induced changes in the direct and indirect gap energies. For monolayer MoS 2 , the indirect gap (K-Γ) is higher in energy than the direct gap at K-valley (Fig. 1g ) [20] , [21] , [22] . Since the K-Γ indirect gap ( E KΓ ) reduces with tensile strain faster than the K-K direct gap ( E KK ) [11] , [15] , [16] , [17] , the direct and indirect exciton states will be brought closer in energy by tensile strain, leading to a marked change in direct exciton population and hence the PL intensity. We analyze the steady-state PL intensity by modeling the exciton populations in a simple two-level system (Supplementary Fig. 1 and Supplementary Note 1 ). In thermal equilibrium, the populations of direct N X,D and indirect N X,I excitons follow the Boltzmann distribution N X,I = N X,D exp(−Δ/ k B T ), and 
    N_X,D = N_0/exp( - Δ/k_ BT) + 1,
 (1) where Δ = E X,I − E X,D is the energy difference between the indirect ( E X,I ) and direct ( E X,D ) exciton energies (Fig. 1h ), and N 0 = N X,D + N X,I is the total exciton population. The energy difference Δ is strain dependent, which can be expressed as \(\Delta = ( {E_{{\rm{X}},{\rm{I}}}^0 + {\rm{\delta }}{E_{{\rm{X}},{\rm{I}}}}} ) - ( {E_{{\rm{X}},{\rm{D}}}^0 + {\rm{\delta }}{E_{{\rm{X}},{\rm{D}}}}} ) = {\Delta _0} + (\gamma - 1)\delta {E_{{\rm{X}},{\rm{D}}}}\) , where \(E_{{\rm{X}},{\rm{D}}}^0\) and \(E_{{\rm{X}},{\rm{I}}}^0\) (δ E X,D and δ E X,I ) are the unstrained (strain-induced changes in) energies of the direct and indirect excitons, respectively, \({\Delta _0} = E_{{\rm{X}},{\rm{I}}}^0 - E_{{\rm{X}},{\rm{D}}}^0\) is the unstrained value of Δ, and γ = δ E X,I /δ E X,D , which is related to the ratio of deformation potential of the K-Γ and K-K quasiparticle gaps. The strain-induced shift in the direct exciton energy, i.e., \({\rm{\delta }}{E_{{\rm{X}},{\rm{D}}}} = {E_{{\rm{X}},{\rm{D}}}} - E_{{\rm{X}},{\rm{D}}}^0\) , can be obtained from the difference between PL peak energies of strained and unstrained monolayer MoS 2 . In our analysis, we assumed the PL peak energy of transferred MoS 2 monolayers on sapphire substrates (1.881 eV; vertical line in Fig. 1f ) as the direct exciton energy of unstrained monolayer MoS 2 (Supplementary Fig. 2 ). By fitting Eq. ( 1 ) to the experimental data and considering Δ 0 and γ as fitting parameters, we obtain a very good fit (solid curve in Fig. 1f ) and determine Δ 0 = 0.08 eV and γ = 1.95 ± 0.14 (see Supplementary Figs. 3 and 4 ), indicative of a direct optical gap in unstrained MoS 2 monolayer, consistent with past understandings [7] , [8] , [20] , [21] , [22] . PL inhomogeneity in strained MoSe 2 –WSe 2 lateral HJs We now turn to the study of strained WSe 2 . 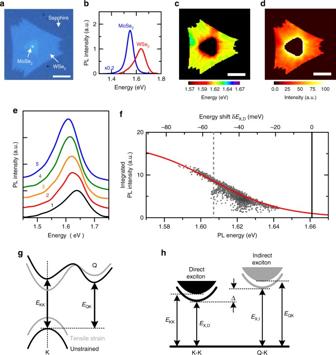Fig. 2 PL inhomogeneity in strained MoSe2–WSe2lateral HJs.aOptical image of a monolayer MoSe2–WSe2HJ.bThe PL spectra of the inner MoSe2and the outer WSe2.c,dContour color maps of the PL peak energy (c) and intensity (d) of outer WSe2.eFive selected PL spectra from the outer WSe2. (f) Integrated PL intensity as a function of peak energy (black dots). Solid line is the model fitting curve. The top axis is the PL peak energy shift with respect to the unstrained WSe2.gSchematics for the band structures of monolayer WSe2without (black) and with (gray) tensile strain.hSchematics for the direct (K-K) and indirect (Q-K) excitonic states with energies ofEX,DandEX,I, respectively Figure 2a shows the optical image of a typical MoSe 2 –WSe 2 lateral HJs, where the inner and outer regions have been identified as MoSe 2 and WSe 2 monolayers, respectively, by PL measurements (Fig. 2b ). As shown in the spatially resolved PL measurements (Fig. 2c, d ) and the selected PL spectra from different areas (Fig. 2e ), the outer WSe 2 region also exhibits remarkable variations in local PL intensity and energy due to the spatial strain inhomogeneity. Since the lattice mismatch between MoSe 2 and WSe 2 is small (<0.2%) [23] , the strain inhomogeneity is likely to arise from the cooling process after high-temperature growth owing to the mismatch in thermal expansion coefficients between TMDs and substrates [24] , [25] , [26] , [27] . In contrary to strained MoS 2 , the PL intensity and energy of the strained WSe 2 shows a “negative” correlation, i.e., the site with a higher PL energy exhibited a lower PL intensity (Fig. 2f ). The negative intensity–energy correlation suggests that the strain-induced change in the indirect gap is very different from that in MoS 2 . In monolayer WSe 2 (Fig. 2g ), the Q-K indirect gap is very close to K-K direct gap. Under tensile strain, the K-K direct gap reduces, while the Q-K indirect gap increases [18] , leading to the increasing PL intensity with tensile strain. Fig. 2 PL inhomogeneity in strained MoSe 2 –WSe 2 lateral HJs. a Optical image of a monolayer MoSe 2 –WSe 2 HJ. b The PL spectra of the inner MoSe 2 and the outer WSe 2 . c , d Contour color maps of the PL peak energy ( c ) and intensity ( d ) of outer WSe 2 . e Five selected PL spectra from the outer WSe 2 . ( f ) Integrated PL intensity as a function of peak energy (black dots). Solid line is the model fitting curve. The top axis is the PL peak energy shift with respect to the unstrained WSe 2 . g Schematics for the band structures of monolayer WSe 2 without (black) and with (gray) tensile strain. h Schematics for the direct (K-K) and indirect (Q-K) excitonic states with energies of E X,D and E X,I , respectively Full size image We use the same model to analyze the PL intensity–energy correlation of strained WSe 2 , but now the indirect exciton represent that formed at the Q-K indirect gap (Fig. 2h ). We have also determined \(E_{{\rm{X}},{\rm{D}}}^0 = 1.661\,{\rm{eV}}\) for unstrained monolayer WSe 2 (vertical line in Fig. 2f ) according to PL measurements on transferred WSe 2 monolayers (Supplementary Fig. 2 ). As shown by the solid curve in Fig. 2f , the model fits the data very well, yielding Δ 0 = −0.07 eV and γ = −0.32 ± 0.05 (Supplementary Fig. 5 ). Interestingly, both Δ 0 and γ for monolayer WSe 2 are negative, in stark contrast to monolayer MoS 2 . The negative γ arises from the opposite energy evolutions of Q and K valleys with strain [18] , while the negative Δ 0 is a direct evidence of indirect optical gap in unstrained monolayer WSe 2 . The indirect gap of monolayer WSe 2 also manifested itself in the large variation in PL intensity (up to a factor of ~ 5) shown in Fig. 2f , because, according to Eq. ( 1 ), the increase in PL intensity by tensile strain should be less than a factor of two if monolayer WSe 2 is initially a direct gap material. Calculated strain-induced bandgap shifts in MoS 2 and WSe 2 monolayers Band structure calculations based on density functional theory (DFT) have been performed and compared to our experimental results. As shown in Fig. 3a , the calculated band structure for unstrained monolayer MoS 2 exhibits a direct gap at the K valleys. The calculated energies of the K-K and K-Γ gaps as a function of strain (Fig. 3c ) show a faster decrease in E KΓ with tensile strain than E KK . If we ignore the strain-induced change in exciton binding energy, the ratio of strain-induced changes in the K-Γ and K-K gaps (i.e., δ E KΓ /δ E KK ) thus represents the ratio of strain-induced changes in the optical gaps γ = δ E X,I /δ E X,D . From the calculations, we determine δ E KΓ /δ E KK = 2.13, consistent with our experimentally obtained γ = 1.95 ± 0.14 for monolayer MoS 2 . On the contrary, our calculations show that unstrained monolayer WSe 2 exhibits an indirect gap between the Q-valley in the CB and the K point in the valence band (VB), as shown in Fig. 3b . Applying tensile strain (Fig. 3d ) tends to shrink the K-K gap, but expand the Q-K gap. We determine δ E QK /δ E KK = −0.28, in good agreement with our experimental value of γ = −0.32 ± 0.05 for monolayer WSe 2 . Fig. 3 DFT calculations of strained MoS 2 and WSe 2 monolayers. a , b The calculated band structures for monolayer MoS 2 ( a ) and WSe 2 ( b ) based on DFT. E KK and E KΓ ( E QK ) denote the direct and the indirect gaps in MoS 2 (WSe 2 ), respectively. c , d Strain-induced energy shifts in the direct and indirect gaps in monolayer MoS 2 ( c ) and WSe 2 ( d ). The calculations show that unstrained WSe 2 is an indirect gap material, which can be turned into a direct-gap material by applying tensile strain Full size image We emphasize that the experimentally determined Δ 0 does not reflect the actual energy difference between the direct and indirect quasiparticle gaps. Due to the strong exciton binding energy caused by reduced dielectric screening in monolayer TMDs [6] , [28] , [29] , the difference in binding energies of direct and indirect excitons has to be taken into account. We first calculate the direct exciton binding energy E B,D based on the effective 2D Coulomb potential (Supplementary Fig. 6 and Supplementary Note 2 ). The indirect exciton binding energy E B,I is then estimated by scaling with the effective reduced masses deduced from band structure calculations. We obtain E B,D = 0.23 eV (K-K) and E B,I = 0.26 eV (K-Γ) for monolayer MoS 2 . The higher E B,I by 0.03 eV, originating from the heavier hole effective mass at Γ-valley, implies that the experimentally determined Δ eV = 0.08 eV underestimates the actual energy difference between the K- and Γ-valleys in the VB, yielding Δ K−Γ = E KΓ − E KK ≈0.11 eV, in good agreement with the value in the range of 0.13–0.30 eV determined by angle-resolved photoemission spectroscopy [20] , [21] , [22] . For monolayer WSe 2 , due to the similar effective mass of electrons at K- and Q-valleys in the CB, the deduced E B,D = 0.19 eV (K-K) and E B,I = 0.20 eV (Q-K) are also similar, yielding Δ K−Q = E QK − E KK ≈−0.06 eV. It demonstrates that monolayer WSe 2 exhibits not only an indirect optical gap, but also an indirect quasiparticle gap with a CB minimum at the Q-valley, which is ~ 60 meV lower than the K-valley, consistent with STS measurements [14] . Temperature dependence of PL intensity–energy correlation We noted that the direct exciton populations in the simple two-level model depend sensitively on temperature. To attest the validity of our model analysis, we have performed the same measurements of spatial PL mapping on another MoSe 2 –WSe 2 HJ flake at T = 150 and 300 K, as shown in Fig. 4a–d . The corresponding PL intensity–energy correlations of the outer monolayer WSe 2 at 150 and 300 K are shown in Fig. 4e . Apart from a rigid shift in PL energy, the PL intensity measured at T = 150 K exhibits a sharper change with energy due to the reduced thermal energy k B T at a lower temperature. The simple two-level model can fit the two data sets with the same Δ 0 and γ -values (solid curves in Fig. 4e ) by simply changing the sample temperature and the unstrained PL peak energy. The temperature dependent measurements thus further confirm that the observed PL intensity–energy correlation is governed by the interplay of direct and indirect exciton populations. The nonuniform distribution of nonradiative defects or inhomogeneous alloy mixing can thus be excluded from the origin of the observed PL intensity–energy correlation. Fig. 4 PL intensity–energy correlations at different temperatures. a – d Contour color maps of PL intensity ( a , c ) and peak energy ( b , d ) in the WSe 2 region of a MoSe 2 –WSe 2 lateral HJ measured at different temperatures: ( a , b ) T = 150 K and ( c , d ) T = 300 K. e Integrated PL intensity as a function of peak energy measured at 150 K (blue dots) and 300 K (red dots). Black lines are model fitting curves Full size image In our analysis, we neglect the influence of dark exciton states at K valleys arising from the spin splitting in the CB. In particular, the spin-forbidden K-K dark exciton state is lower in energy by ~ 30 meV in monolayer WSe 2 [30] , which also affects the bright (direct) exciton populations and hence the PL intensity at different temperatures. However, because the strain-induced change in the CB spin splitting is very small (<0.5 meV/%) [31] , including the dark exciton states will not change the analysis of Δ 0 and γ -values from the PL intensity–energy correlation measured at a given temperature. Strain could also impact the radiative lifetime and the binding energy of the K-K direct exciton through modifications in wave functions, optical matrix element and band curvatures. However, according to the range of PL shifts in our samples and recent theoretical calculations [32] , we estimated that the strain-induced changes in the radiative lifetime and the binding energy are small (<5%), which is within our experimental uncertainty. Spatial variation of the unintentional doping in the sample could also lead to PL shifts due to the charged exciton (trion) emissions. We have performed line-shape analysis for the selected PL spectra shown in Fig. 2e and found that no spectral signature can be attributed to the trion emissions (Supplementary Fig. 7 ). Therefore, spatial variation in doping level can be excluded from the observed PL shift and the intensity–energy correlation. Alloy inhomogeneity caused by material intermixing could be another source of the observed PL inhomogeneity. We have measured the PL inhomogeneity for HJ flakes after ultrasonic treatments. Interestingly, we found that the spatial distributions of PL intensity and energy are changed, but still exhibit a similar negative correlation (Supplementary Fig. 8 ). Since the strain inhomogeneity is likely to form during the fast-cooling process caused by the contraction mismatch, the local interactions between TMD and the substrate could be loosen and redistributed by ultrasonic treatments, and thereby changing the pattern of strain inhomogeneity. This result thus excludes the possibility that the PL inhomogeneity is caused by local variation of doping, defect distribution or alloy composition, since they are unlikely to be altered by ultrasonic treatments. The indirect optical gap in unstrained monolayer WSe 2 identified in this work has important implications. As a light emitter, monolayer WSe 2 is far from ideal as compared with other MX 2 with a direct gap, since a majority of photogenerated carriers will form indirect excitons even at room temperature, which considerably limits the quantum yield of light emissions. On the other hand, the efficient light absorption through the direct optical gap, together with the suppressed radiative recombination efficiency for the indirect excitons, makes monolayer WSe 2 very ideal for photovoltaic applications. The indirect Q-K exciton in WSe 2 is essentially dark and inaccessible optically. Recent theoretical work predicted that non-covalently attached molecules with a strong dipole moment can turn the indirect dark exciton bright, implicating its applications in molecule sensing [33] . Nevertheless, applying a moderate tensile strain (~ 1% uniaxial or ~ 0.5% biaxial) can tune the bandgap from indirect to direct, which can improve drastically the emission efficiency by nearly an order of magnitude. 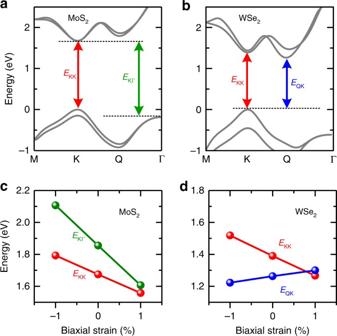Fig. 3 DFT calculations of strained MoS2and WSe2monolayers.a,bThe calculated band structures for monolayer MoS2(a) and WSe2(b) based on DFT.EKKandEKΓ(EQK) denote the direct and the indirect gaps in MoS2(WSe2), respectively.c,dStrain-induced energy shifts in the direct and indirect gaps in monolayer MoS2(c) and WSe2(d). The calculations show that unstrained WSe2is an indirect gap material, which can be turned into a direct-gap material by applying tensile strain 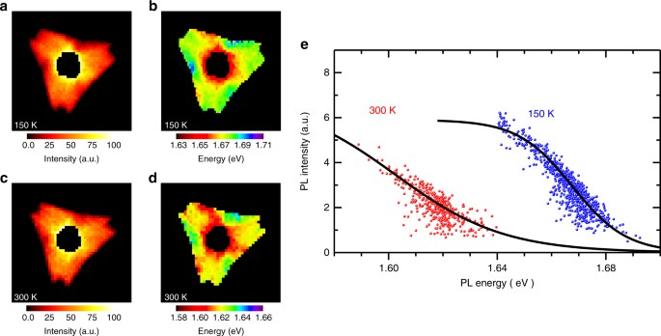Fig. 4 PL intensity–energy correlations at different temperatures.a–dContour color maps of PL intensity (a,c) and peak energy (b,d) in the WSe2region of a MoSe2–WSe2lateral HJ measured at different temperatures: (a,b)T= 150 K and (c,d)T= 300 K.eIntegrated PL intensity as a function of peak energy measured at 150 K (blue dots) and 300 K (red dots). Black lines are model fitting curves Based on the simple two-level model, we estimated that the crossover of the direct and indirect optical gaps occurs at 1.607 eV (1.797 eV) for monolayer WSe 2 (MoS 2 ), as indicated by the vertical dash line in Fig. 2f (Fig. 1f ). For the strained MoSe 2 –WSe 2 lateral HJs investigated here, the PL peak energy of the WSe 2 region spans from 1.58 to 1.64 eV, which covers the crossover energy of direct and direct optical gap at 1.607 eV. This means that local strain variation also gives rise to a spatial modulation of direct and indirect gap, which forms a very unique platform with nonuniform potential modulations for studying exciton diffusions and localizations. Finally, we point out that the indirect gap nature of monolayer WSe 2 must to be taken into account in further studies of its fundamental properties (e.g., exciton spin valley dynamics) and device applications for light emissions and harvesting. Growth of monolayer lateral heterojunctions High-quality single-crystal TMD HJs were synthesized on sapphire substrates by chemical vapor deposition (CVD) in horizontal hot-wall chambers. The monolayer WSe 2 –MoS 2 lateral HJs were grown using the two-step growth method (see ref. [19] for details), while MoSe 2 –WSe 2 lateral HJs were grown using the conventional one-pot synthesis process. For WSe 2 –MoS 2 HJs, we used high-purity WO 3 , MoO 3 , Se and S powders as the source precursors. The growth temperatures for WSe 2 and MoS 2 are 925 and 755°C, respectively. For MoSe 2 –WSe 2 HJs, high-purity MoO 2 , WO 3 , and Se powder were used as the initial reactants, and the HJs were grown at 880°C. All growths were performed in Ar/H 2 flowing gas at low pressure (5–40 Torr). Optical measurements PL and Raman measurements were performed using a home-built optical microscope in the back-scattering configuration. A 532 nm solid-state laser was used as the excitation source. The laser were focused on the sample by a 100 × objective lens (NA = 0.9). The PL and Raman signals were collected by the same objective, analyzed by a 0.75-m monochromator and detected by a nitrogen-cooled CCD camera. For confocal measurements, the sample image was projected onto a 50 μm pinhole before entering the monochromator, yielding an overall spatial resolution of ~ 0.5 μm. Room temperature spatial mappings of PL spectra were performed using a fast motorized x–y stage with a step size of 0.25 μm. Low-temperature measurements were performed in a cryogen-free and vibration-free cryostat equipped with a 3-axis piezo-positioner, an x-y scanner and an objective lens (N.A. = 0.82) in the low-temperature chamber. DFT calculations The first-principle calculations were based on the generalized gradient approximation (GGA) [34] using the full-potential projected augmented wave method [35] , [36] as implemented in the Vienna ab initio simulation (VASP) package [37] , [38] . The electronic structures of monolayer MoS 2 and WSe 2 were calculated using a 30 × 30 × 1 Monkhorst-Pack k -mesh over the Brillouin zone with a cutoff energy of 500 eV under geometry optimization. The spin-orbit coupling was included in a self-consistent manner. Slabs with vacuum thickness larger than 30 Å were used to model the thin films. For the strain effects, the atomic positions were relaxed until the residual forces were less than 0.001 eV/Å. Data availability The data that support the findings of this study are available from the corresponding author upon reasonable request.